Sequential pH-driven dimerization and stabilization of the N-terminal domain enables rapid spider silk formation The mechanisms controlling the conversion of spider silk proteins into insoluble fibres, which happens in a fraction of a second and in a defined region of the silk glands, are still unresolved. The N-terminal domain changes conformation and forms a homodimer when pH is lowered from 7 to 6; however, the molecular details still remain to be determined. Here we investigate site-directed mutants of the N-terminal domain from Euprosthenops australis major ampullate spidroin 1 and find that the charged residues D40, R60 and K65 mediate intersubunit electrostatic interactions. Protonation of E79 and E119 is required for structural conversions of the subunits into a dimer conformation, and subsequent protonation of E84 around pH 5.7 leads to the formation of a fully stable dimer. These residues are highly conserved, indicating that the now proposed three-step mechanism prevents premature aggregation of spidroins and enables fast formation of spider silk fibres in general. Spider dragline silk, one of the toughest biomaterials known, is produced through the assembly of large proteins (spidroins) with remarkable biochemical properties. The major ampullate spidroin (MaSp) 1 is synthesized in the major ampullate gland and consists of a central ~3,500-residue repetitive region with alternating polyalanine- and glycine-rich segments, flanked by two globular regions: a highly conserved N-terminal (NT) domain and a less conserved C-terminal domain of ~130 and ~110 residues, respectively [1] , [2] . Although spidroins are highly aggregation-prone, they are stored as a soluble dope at concentrations up to 50% (w/w) in the sac of the silk gland [3] , [4] . Spidroins are processed into silk fibres during passage through an elongated duct [5] . At a molecular level, during this phase transition, soluble proteins with mainly helical and random-coil structures convert into insoluble polymers dominated by β-sheets [4] , [6] . This structural transformation is regulated by changes in several environmental factors, including shear forces as the duct gradually narrows [7] and changes in the ion concentration [8] . In addition, spidroins are subjected to a pH drop from ~7 in the middle region of the storage sac to 6.3 in the duct [9] , [10] . Recently, we used concentric ion selective microelectrodes [11] to measure a pH ~5.7 halfway through the major ampullate duct, and the pH likely reaches even lower levels in the distal part of the duct (MA et al ., unpublished work). The MaSp1 NT domain is highly sensitive to changes in pH and is proposed to function as a pH-regulated relay with a dual function: conferring solubility at high pH and facilitating fibre formation at low pH [12] , [13] , [14] . NT is mainly monomeric at pH 7 and dimeric at pH 6 (refs 13 , 14 , 15 ) but the associated molecular mechanisms are still largely unknown. The high-resolution X-ray structure of MaSp1 NT from Euprosthenops australis demonstrates a homodimer, where each subunit adopts a five-helix bundle fold and helix 2, 3 and 5 form the dimer interface. These subunits have a pronounced dipolar character, with positive and negative residues clustered at opposite ends, and arrange in an anti-parallel manner. Seven acidic (D39, D40, E79, E84, E85, E119 and D134) and three basic (H6, R60 and K65) residues constitute the positive and negative pole of the NT subunit, respectively [12] . Using nuclear magnetic resonance (NMR) spectroscopy, it was shown that MaSp NT from Latrodectus hesperus is a monomer at pH 7.2 (ref. 14 ) and a recently solved solution structure of MaSp1 NT from E. australis at pH 7.2 reveals a monomer with distinct structural differences from the dimer subunit [16] . Mainly, helix 3 is significantly shifted, creating a less compact helix bundle that is incompatible with the dimer crystal structure. Notably, the structural rearrangements required for monomer to dimer interconversion include a relocation of the single tryptophan residue (W10) from being buried in the hydrophobic core of the monomer to a more solvent-exposed environment in the dimer [16] . The dimer crystal structure and the monomer NMR structure from E. australis presumably represent the pH 6 and pH 7 conformations, respectively. However, NT crystals were prepared at pH 7, where monomers would be expected. Although up to 1 unit lower pH inside crystals compared with the surrounding buffer has been observed [17] , it is important to question whether the NT crystal structure reflects the fully stable dimer conformation at low pH. It is not established which side chains have p K a values within the pH interval relevant for NT interconversion from a monomer to dimer. Theoretical prediction of titratable residues within a protein is usually complicated as p K a values can be significantly perturbed depending on local environment [18] . Since clustering of acidic residues frequently leads to elevated p K a values [19] , the closely located conserved residues, E79, E84 and D40, were previously investigated. Glu and Asp were exchanged with Gln and Asn, respectively, in the mutants NT D40N , NT E79Q , NT E84Q and the doubly mutated NT D40NE84Q . The non-conserved H6 was also included as a deletion mutant, NT H6 Δ . However, none of the residues alone, or D40 and E84 together, mediate pH sensitivity [12] . Later, electrospray ionization mass spectrometry (ESI-MS) at pH 6 and 7 revealed that NT D40N and NT D40NE84Q were not able to form dimers within this pH interval. However, NT E79Q and NT E84Q dimerized at low pH, although to a limited extent for the latter [15] . A molecular dynamics simulation predicted the p K a values of all ionizable side chains upon dissociation of dimers into monomers [20] . Here E79 and E119 were identified as the only residues with p K a in the relevant pH range. Furthermore, stabilizing intersubunit salt bridges in the dimer could form between D40-K65 and D39-R60 (refs 12 , 20 ). A recent investigation of the dimerization kinetics of single NT mutants showed that only D39N and D40N completely abolished dimerization. E84Q showed only a minor effect and E119Q was the only mutation that significantly stabilized the dimer [21] . Herein, we investigated several new mutants for shifts in monomer–dimer equilibrium using Trp fluorescence spectroscopy. Urea-induced denaturation of the mutants and wild-type (wt) NT was used to calculate the proton exchange between the native dimer and the denatured monomer. Two mutants were also evaluated by ESI-MS, hydrogen-deuterium exchange (HDX)-MS, circular dichroism (CD) and NMR spectroscopy. On the basis of these experiments, we present a three-step mechanism for NT dimerization in which NT monomers (i) associate by electrostatic interactions and (ii) at around pH 6.5 form weakly associated dimers and (iii) close to the silk gland exit point form stable dimers that interconnect the spidroins. This mechanism provides explanations both to how rapid fibre formation is mediated and how precocious aggregation is avoided. NMR structure of wt NT at pH 5.5 compared with X-ray structure On the basis of assignments of the wt NT monomer at pH 7.2 (ref. 16 ), almost complete backbone and side chain assignments of wt NT at pH 5.5 were obtained using interactive analysis of an HNCA and three 3D (three-dimensional) 15 N/ 13 C-resolved nuclear Overhauser enhancement (NOE) spectroscopy (NOESY)-heteronuclear single quantum coherence (HSQC) spectra. Initially, we solved the pH 5.5 structure as a monomer and found that it is very similar to the crystal dimer subunit with a surface-exposed W10 side chain. 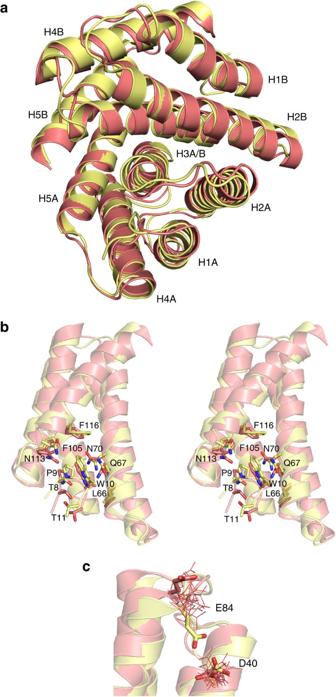Figure 1: Comparison of dimeric wt NT structures. (a) Global superposition of the representative conformer of the wt NT NMR structure at pH 5.5 (pink) and the crystal structure at pH 7.0 (yellow). Secondary structure elements are labelled H1–H5, and the letter A/B indicates the subunit. (b) Stereo view of the superposed NMR and crystal dimer subunits showing side chain orientations within 5 Å around the residue W10. (c) Close-up view of side-chain orientations of residues D40 and E84 that form a handshake interaction in the crystal dimer structure. Side chains of the other 19 conformers of the NMR structure are shown with thin lines. In (a–c) the structures were superimposed for minimal RMSD of the backbone N, Cαand C′ atoms of residues 8–82 and 90–130. The figure was generated using PyMOL38. Additionally, RPF scores [22] ( Supplementary Table 1 ) reflecting the goodness-of-fit of a structure to the NMR data indicated that the crystal dimer fits very well with the NOESY data at pH 5.5. In order to verify that NT is dimeric at pH 5.5, we performed 15 N NMR relaxation measurements sensitive to motions on a pico- to nanosecond timescale. Model-free analysis of the relaxation data ( Supplementary Fig. 1 ) yielded overall molecular tumbling correlation times of 15.6 ns at pH 5.5 consistent with the molecular weight expected for a dimer (29.8 kDa), and 8.8 ns at pH 7.2 consistent with a monomer (14.9 kDa), respectively. Encouraged by this and the close similarity of the initial structure to the dimer subunit crystal structure, we then inspected NOESY spectra for intermolecular contacts observed in the crystal dimer. In total, 19 unambiguous unique intermolecular contacts were established ( Supplementary Fig. 2 ) and used as distance constraints for refinement of the crystal structure against solution NOESY data. This approach was used to reduce the assignment ambiguity during automated NOE assignment and structure calculation, and resulted in a high-quality NMR structure with improved RPF scores, as shown by the statistics for the final 20 NMR conformers ( Supplementary Table 1 ). The NMR structure at pH 5.5 is very similar to the crystal structure at pH 7.0 ( Fig. 1a ), with an RMSD of 1.15 Å calculated for the backbone atoms of both chains (residues 8–82, 90–130). In the two dimer structures, all helices are in the same orientation and the conformation of side chains constituting the dimer interface mostly coincide. Basic and acidic residues on the opposite ends of the dimer subunit are positioned similarly and a salt bridge between D40 and K65 is present in both structures. Moreover, in both structures M132 from the C-terminus of one subunit packs into a crevice near the N-terminus of the other subunit. These observations were verified by manual inspection of the expected intermolecular NOEs. Notably, both structures also feature a highly similar side chain arrangement near W10 ( Fig. 1b ), which is central to the monomer–dimer interconversion [16] . A distinct feature of the newly determined NMR structure is the absence of the D40-E84 intramolecular ‘handshake interaction’: in all 20 NMR conformers the oxygen atoms of the side chain carboxylates are more than 8 Å apart ( Fig. 1c ). This may be due to increased mobility of the loop between H3 and H4 (see relaxation analysis in Supplementary Fig. 1 ) that includes E84; however, we cannot exclude that the absence of this interaction is a consequence of a lack of NMR restraints as the nearest protons from these two side chains in the crystal structure are about 6 Å apart. Figure 1: Comparison of dimeric wt NT structures. ( a ) Global superposition of the representative conformer of the wt NT NMR structure at pH 5.5 (pink) and the crystal structure at pH 7.0 (yellow). Secondary structure elements are labelled H1–H5, and the letter A/B indicates the subunit. ( b ) Stereo view of the superposed NMR and crystal dimer subunits showing side chain orientations within 5 Å around the residue W10. ( c ) Close-up view of side-chain orientations of residues D40 and E84 that form a handshake interaction in the crystal dimer structure. Side chains of the other 19 conformers of the NMR structure are shown with thin lines. In ( a – c ) the structures were superimposed for minimal RMSD of the backbone N, C α and C′ atoms of residues 8–82 and 90–130. The figure was generated using PyMOL [38] . Full size image Design of E. australis MaSp1 NT mutants In order to identify the key residues involved in dimer formation, we further evaluated the previously described NT D40N , NT E79Q , NT E84Q and NT D40NE84Q (ref. 12 ) together with a novel set of mutants. E79, E84 and E119 were substituted with Gln in different combinations to give NT E119Q , NT E79QE119Q and NT E79QE84Q . Encouraged by early results (see below), we subsequently designed the triple mutants NT E79QE84QE119Q , NT D40NE79QE119Q and NT H6AE79QE119Q . K65 and R60 are not expected to have p K a values close to the monomer–dimer transition point but are predicted to stabilize the dimer by salt-bridge formation between the subunits [20] . An interaction between K65–D40 was observed in most NMR conformers at pH 5.5. To further investigate how electrostatic interactions contribute to the formation of stable dimers, K65 and R60 were substituted with Ala in NT K65A and NT R60A . In addition, the consequence of introducing repelling charges between the subunits, as opposed to a salt bridge, was examined by replacing K65 with Asp (NT K65D ) or D40 with Lys (NT D40K ). We also studied NT A72R , for which NMR and X-ray structures revealed a constitutive monomer between pH 7.5 and 5.5, with a conformation very similar to the NMR structure of wt NT at pH 7.2 (ref. 16 ). Dimerization analysis of NT mutants Trp fluorescence spectra were measured at pH 5.6–7.4 for wt NT and all mutants. The results are expressed as the ratio between the fluorescence at 339 and 351 nm, which reflects the ratio between monomeric and dimeric NT [16] . Since the presence of NaCl stabilizes the monomer conformation [13] , [14] , measurements were made without salt as well as at a physiological concentration (154 mM). Similar shifts in Trp fluorescence ratios were observed when NaCl was substituted with Na 2 SO 4 or NaNO 3 ( Supplementary Fig. 3 ), which indicates that the behaviour of wt NT in the presence of NaCl can be attributed to general salt effects. Importantly, the same monomer to dimer interconversion as seen for NT occurs in a construct where NT is linked to five polyalanine/glycine-rich co-blocks (NT-5Rep), which mimics its native situation in spidroins ( Supplementary Fig. 4 ). The wt NT shows sigmoidal behaviour with a transition point around pH 6.5 for the monomer–dimer equilibrium in the absence of NaCl ( Fig. 2a ) and around 6.0 in the presence of 154 mM NaCl ( Supplementary Fig. 5 ). As expected [16] , the NT A72R mutant favours the monomer conformation at all pH values ( Fig. 2b ). Trp fluorescence data for several of the acidic-residue mutants show significantly shifted transition points in the absence of salt compared with wt NT ( Fig. 2a ). A decrease in the apparent p K a of dimerization to 5.9 and 5.6 is observed for NT D40N and NT D40NE84Q , respectively, while NT E84Q shows only a slight decrease in p K a of dimerization. These results support the previous finding [12] and indicate the importance of D40, either for a charge clustering interaction with E84 and/or for an intersubunit salt-bridge formation with K65. The mutants NT E79Q and NT E119Q were the only single mutants observed to favour the dimer conformation compared with wt NT. The p K a of dimerization increased to 6.8 for NT E79Q and is estimated to be ~7.5 for NT E119Q since a stable monomeric state is not reached within the measured pH range ( Fig. 2a ). The double mutant NT E79QE119Q demonstrated a synergetic effect with a very low amount of monomers present at high pH. This suggests that E79 and E119 become protonated upon dimerization. A small difference in the Trp fluorescence ratio between pH 5.6 and pH 7.4 ( Fig. 2a ) (and HSQC NMR spectra, see below), however, led to the conclusion that protonation of at least one additional residue was required for stable dimer formation. 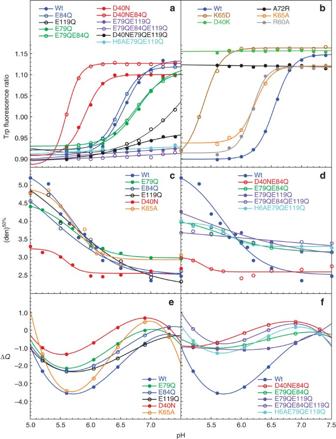Figure 2: Dimerization analysis and stability measurements of NT mutants. (a,b) Trp fluorescence ratio of NT mutants and wt NT as a function of pH, measured in 20 mM HEPES/20 mM MES buffer for (a) acidic residue mutants and (b) basic residue mutants. To clarify the shift in Trp fluorescence observed after addition of E84Q, the same colour with filled and open circles, respectively, was chosen for wt NT and E84Q (blue), E79Q and E79QE84Q (dark green), E79QE119Q and E79QE84QE119Q (purple) as well as for D40N and D40NE84Q (red). The solid line represents the equation from fitting the data to a two-state binding model and the results are representative of more than three experiments. (c,d) Urea-induced denaturation of NT mutants and wt NT in the presence of 0–7 M urea, measured with Trp fluorescence and presented as transition points between native and denatured states ([den]50%) as a function of pH for (c) single mutants and (d) double and triple mutants. (e,f) Calculated differences in charge (ΔQ) between the native and denatured states for (e) single mutants and (f) double and triple mutants. Figure 2: Dimerization analysis and stability measurements of NT mutants. ( a , b ) Trp fluorescence ratio of NT mutants and wt NT as a function of pH, measured in 20 mM HEPES/20 mM MES buffer for ( a ) acidic residue mutants and ( b ) basic residue mutants. To clarify the shift in Trp fluorescence observed after addition of E84Q, the same colour with filled and open circles, respectively, was chosen for wt NT and E84Q (blue), E79Q and E79QE84Q (dark green), E79QE119Q and E79QE84QE119Q (purple) as well as for D40N and D40NE84Q (red). The solid line represents the equation from fitting the data to a two-state binding model and the results are representative of more than three experiments. ( c , d ) Urea-induced denaturation of NT mutants and wt NT in the presence of 0–7 M urea, measured with Trp fluorescence and presented as transition points between native and denatured states ([den] 50% ) as a function of pH for ( c ) single mutants and ( d ) double and triple mutants. ( e , f ) Calculated differences in charge (Δ Q ) between the native and denatured states for ( e ) single mutants and ( f ) double and triple mutants. Full size image Given that E84 is the only remaining well-conserved acidic residue [23] , [24] , we evaluated the triple mutant NT E79QE84QE119Q . Although protonation of D40 as analysed by the mutant NT D40N strongly stabilizes the monomer ( Fig. 2a ), the triple mutant NT D40NE79QE119Q was included to rule out any synergetic effects. NT H6AE79QE119Q was also evaluated to verify that H6 does not contribute to the pH sensitivity [12] . Our measurements show that NT H6AE79QE119Q does not significantly differ from NT E79QE119Q , and confirms that the non-conserved H6 does not contribute to dimer formation. NT D40NE79QE119Q stabilizes the monomer conformation compared with NT E79QE119Q , which further confirms that D40 does not take part in the protonation events. In contrast, NT E79QE84QE119Q stabilizes the dimer conformation compared with NT E79QE119Q and the Trp fluorescence ratio is close to what would be expected from a constitutive dimer ( Fig. 2a ). In the presence of NaCl ( Supplementary Fig. 5a ), the monomer conformations are generally highly stabilized. However, the p K a of dimerization observed for the mutants relative to wt NT are comparable to those measured without salt. Hence, the fluorescence ratios in the presence of NaCl support the conclusions drawn from the ratios in the absence of salt. ESI-MS of NT E79QE119Q and NT E79QE84QE119Q at pH 5.5 and pH 7.5 show pH-independent dimerization ( Supplementary Fig. 6 ). Analysis with HDX-MS shows that the central segment of helix 3 in wt NT is protected from H/D exchange at pH 5.5 but not at 7.5 (ref. 15 ). When analysing the two mutants, the segment is protected from H/D exchange at both pH 5.5 and 7.5 ( Supplementary Fig. 7 ). The p K a of dimerization of the basic residue mutants NT K65A and NT R60A are shifted down from pH 6.5 to around pH 6.2 for both variants ( Fig. 2b ), and a similar relative shift is observed in the presence of NaCl ( Supplementary Fig. 5b ). These data support the hypothesis that intermolecular salt bridges contribute but are not essential for dimer formation. However, due to the close proximity of D39 and D40 with K65 and R60, a single point mutation may be counteracted by the formation of compensatory salt bridges. Therefore, it cannot be ruled out that the importance of electrostatic interactions is underestimated by analyses of NT K65A and NT R60A single mutants. NT K65D and NT D40K highly favour the monomer conformation ( Fig. 2b ). NT K65D only begins to dimerize at very low pH, with a p K a of dimerization estimated to be around 5.2–5.3. However, NT D40K exclusively forms monomers in the entire pH range. In the presence of NaCl, both mutants behave strictly as monomers with fluorescence ratios comparable to NT A72R ( Supplementary Fig. 5b ). Proton uptake for native and denatured dimer For the association of wt NT from monomers to dimers between pH 7.5 and 5.5, as measured by Trp fluorescence ratio, we assume the following reaction to occur: where B is monomeric protein, n is the number of protons that exchange during the pH titration and K a is the apparent acid dissociation constant. The process is independent of protein concentration from 10 μM to 1 mM ( Supplementary Fig. 8 ). We analyse the data at the monomer level as a simple association of protons, and this gives rise to the following equation: where F is the measured fluorescence and F B and F BH are the fluorescence values of the non-protonated and protonated species, respectively. By analysing the Trp fluorescence data for wt NT ( Fig. 2a ) using equation (2), we estimate that on average 3.22 (±0.19) protons are taken up by each monomer unit over the pH range 7.5–5.5. In addition, the stability of wt NT and individual NT mutants was determined by urea-induced denaturation for subsequent analysis of the proton uptake. The Trp fluorescence ratio was measured in the presence of 0–7 M urea at constant pH values ranging from 5.0 to 7.5. For each measured pH, the concentration at which the protein is 50% denatured ([den] 50% ) was determined from plots of the fluorescence ratio against the urea concentration. The [den] 50% were then plotted as a function of pH to obtain a measure of the stability of individual NT mutants ( Fig. 2c,d ). On the basis of protein-folding theory (see Methods), we calculated the difference in charge between the native and denatured states as a function of pH between pH 5.0 and 7.5 ( Fig. 2e,f ). According to Fig. 2e,f , the maximal proton uptake—that is, the difference between native dimer and denatured monomer—is 3.6 for wt NT. This is very similar to the proton uptake associated with dimerization—that is, the difference between native dimer and native monomer, as calculated from Trp fluorescence data (above). This leads us to conclude that the native monomer and the denatured monomer have approximately the same number of protons bound. Thus, each dimer subunit takes up approximately three protons compared with the monomer, and these protons are then released upon denaturation. We would predict that the mutants that have fewer protons taken up due to dimerization would also have a smaller difference in charge between native dimer and denatured monomer. In fact, the single mutants NT E84Q , NT E79Q and NT E119Q lose 1.3, 1.4 and 1.3 protons, respectively, compared with wt NT ( Fig. 2e ). The charge differences appear to be additive as the double mutants NT E79QE84Q and NT E79QE119Q show a loss of 2.6 and 2.5 protons, respectively, and the triple mutant NT E79QE84QE119Q shows a loss of 2.9 protons ( Fig. 2f ). The triple mutant NT H6AE79QE119Q has a similar proton uptake compared with that of NT E79QE119Q confirming that H6 does not contribute by protonation. We also observed a significant charge reduction for NT D40N , which loses 2.2 protons ( Fig. 2e ). The wt NT has a monomer–dimer p K a of around 6.5 ( Fig. 2a ) but the greatest proton difference between the native and denatured state occurs around pH 5.7 ( Fig. 2e ). This indicates that upon lowering of pH, NT first dimerizes and subsequently gets stabilized (see below and Fig. 7 ). The mutants NT E119Q and NT K65A have their p K a values shifted +0.6 and −0.3, respectively, but the greatest proton difference also occurs around pH 5.7. NT E79QE119Q also has a strongly shifted p K a , which cannot be determined clearly but is >>7, and has a shallow maximum proton uptake around pH 5.8–6, further supporting that the monomer–dimer p K a as measured by Trp fluorescence reflects another process than stability of the native state as measured by urea denaturation (see further under Discussion below). Figure 7: Proposed mechanism for NT dimerization. ( a ) NT molecules with a monomer conformation where W10 is buried in the hydrophobic core. ( b ) Electrostatic interactions mediated by D40, K65 R60 and possibly E84 in their charged state lead to elevated p K a values for E79 and E119 due to a changed environment between associated monomer subunits. ( c ) Protonation of E79 and E119 at pH 6.5 leads to the structural conversion to a weakly associated dimer conformation in which W10 becomes exposed to a more polar environment. 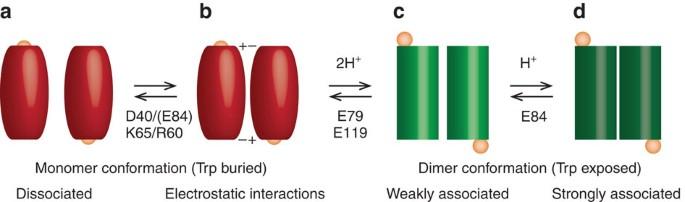Figure 7: Proposed mechanism for NT dimerization. (a) NT molecules with a monomer conformation where W10 is buried in the hydrophobic core. (b) Electrostatic interactions mediated by D40, K65 R60 and possibly E84 in their charged state lead to elevated pKavalues for E79 and E119 due to a changed environment between associated monomer subunits. (c) Protonation of E79 and E119 at pH 6.5 leads to the structural conversion to a weakly associated dimer conformation in which W10 becomes exposed to a more polar environment. (d) Upon further decrease in pH to 5.7, protonation of E84 promotes conversion from weakly associated dimers to strongly associated and fully stable dimers. ( d ) Upon further decrease in pH to 5.7, protonation of E84 promotes conversion from weakly associated dimers to strongly associated and fully stable dimers. Full size image HSQC NMR spectra of NT E79QE119Q and NT E79QE84QE119Q Assuming that a constitutive dimer will maintain its structure under conditions where wt NT would form mainly monomers—that is, at pH 7 and above—we evaluated the structural similarity between the mutants NT E79QE119Q and NT E79QE84QE119Q at pH 7.2 and the wt NT dimer at pH 5.5 using two-dimensional (2D) HSQC NMR spectroscopy. The 2D HSQC spectrum of NT E79QE119Q recorded at pH 7.2 shows two sets of peaks indicating the presence of two conformations that are in slow exchange on the NMR timescale ( Fig. 3a ). Both sets have HSQC fingerprints more similar to the wt NT dimer than the monomer; however, neither one seems to represent the wt-like dimer as a pH change to 5.5 yields a different spectrum with one set of peaks that is almost identical to the spectrum of wt NT at pH 5.5. In contrast, the 2D HSQC spectrum of NT E79QE84QE119Q at pH 7.2 is similar to the spectrum of wt NT at pH 5.5 and does not change significantly upon reduction of the pH to 5.5 ( Fig. 3b ). Further comparison of backbone amide chemical shifts between NT E79QE84QE119Q at pH 7.2 and wt NT at pH 5.5 reveals only small differences, while significantly larger differences are evident in comparison with the chemical shifts of the wt NT monomer at pH 7.2 ( Fig. 3c ). 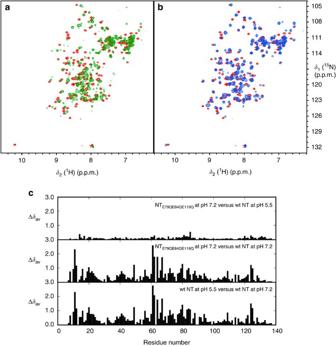In addition, the pattern of NT E79QE84QE119Q chemical shift differences with respect to the wt NT monomer matches that of the wt NT dimer. Figure 3: Comparison of NTE79QE119Qand NTE79QE84QE119Qwith the wt NT dimer using 2D HSQC NMR. (a) Overlay of15N-1H HSQC NMR spectra of NTE79QE119Qat pH 7.2 (green) and wt NT pH 5.5 (red). (b) Overlay of15N-1H HSQC NMR spectra of NTE79QE84QE119Qat pH 7.2 (blue) and wt NT pH 5.5 (red). (c) Averaged backbone amide1H and15N chemical shift differences Δδav=between NTE79QE84QE119Qat pH 7.2, wt NT dimer at pH 5.5 and wt NT monomer at pH 7.2. Figure 3: Comparison of NT E79QE119Q and NT E79QE84QE119Q with the wt NT dimer using 2D HSQC NMR. ( a ) Overlay of 15 N- 1 H HSQC NMR spectra of NT E79QE119Q at pH 7.2 (green) and wt NT pH 5.5 (red). ( b ) Overlay of 15 N- 1 H HSQC NMR spectra of NT E79QE84QE119Q at pH 7.2 (blue) and wt NT pH 5.5 (red). ( c ) Averaged backbone amide 1 H and 15 N chemical shift differences Δ δ av = between NT E79QE84QE119Q at pH 7.2, wt NT dimer at pH 5.5 and wt NT monomer at pH 7.2. Full size image CD spectroscopy of NT E79QE119Q and NT E79QE84QE119Q The spectra recorded at pH 8.0 show a typical behaviour for wt NT [13] , [25] , a mainly α-helical secondary structure at 25 °C and random-coil structure at 95 °C, which is able to refold upon cooling ( Fig. 4a ). Our measurements show a somewhat less helical structure of wt NT after refolding at pH 5.5 compared with at pH 8.0 ( Fig. 4b ). The recorded spectra for the two NT mutants, before denaturation, are very similar to wt NT at both pH values ( Fig. 4c–f ). After thermal denaturation at pH 8.0, both mutants are able to refold to the same extent as wt NT ( Fig. 4 , left panel). However, at pH 5.5, NT E79QE119Q refolds into a structure, lacking the typical spectral characteristics of a mainly α-helical protein ( Fig. 4d ), while NT E79QE84QE119Q remains in an unstructured denatured state with a low CD signal after cooling ( Fig. 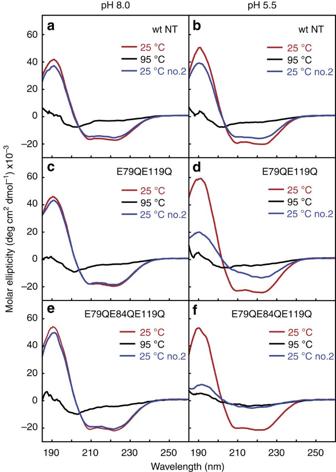4f ). Figure 4: CD spectra of NTE79QE119Qand NTE79QE84QE119Q. The residual molar ellipticity was measured at 25, 95 and 25 °C after cooling for wt NT at (a) pH 8.0 and (b) pH 5.5, NTE79QE119Qat (c) pH 8.0 and (d) pH 5.5 and NTE79QE84QE119Qat (e) pH 8.0 and (f) pH 5.5. The data are presented as smoothed averages of four measurements. Figure 4: CD spectra of NT E79QE119Q and NT E79QE84QE119Q . The residual molar ellipticity was measured at 25, 95 and 25 °C after cooling for wt NT at ( a ) pH 8.0 and ( b ) pH 5.5, NT E79QE119Q at ( c ) pH 8.0 and ( d ) pH 5.5 and NT E79QE84QE119Q at ( e ) pH 8.0 and ( f ) pH 5.5. The data are presented as smoothed averages of four measurements. Full size image The melting temperature ( T m ) was estimated from the transition point between the folded and denatured states. As expected from the formation of stable dimers for wt NT upon lowering of pH, we observed a significantly increased T m from 54 °C at pH 8.0 to 65 °C at pH 5.5 ( Fig. 5a,b ). The wt NT monomer at pH 7.2 is sensitive to salt-screening, showing an increased thermal stability with an increased concentration of salt due to shielding of negative and positive charge clusters [14] . Hence, the pH-dependent difference in T m for wt NT can, in addition to increased stability of the dimer conformation relative to the monomer conformation, be attributed to the presence of destabilizing intramolecular repelling charge clusters D39/D40 and R60/K65 in the monomer, which become neutralized by formation of intermolecular salt bridges between D39 and K60 and D40 and K65, respectively, in the dimer. We show that the two mutants are remarkably more stable than wt NT at pH 8.0 with a T m identical to the wt NT at pH 5.5. 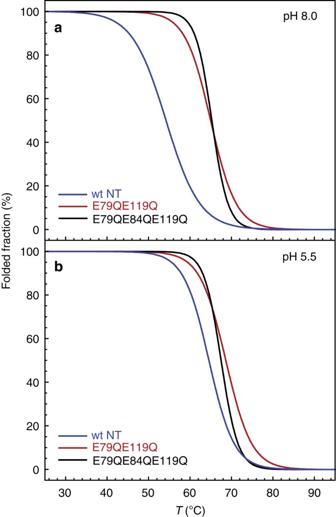Upon lowering the pH, the T m for the mutants only slightly increases to 69 °C and 68 °C for NT E79QE119Q and NT E79QE84QE119Q , respectively. Figure 5: Temperature-induced unfolding of NTE79QE119Qand NTE79QE84QE119Q. The CD signal was measured at 222 nm and converted to fraction folded according to the formula ([CD]obs–[CD]D)/([CD]N–[CD]D), where CD is the signal measured in mdegrees, CDD is the signal for the denatured state, CDN is the signal for the native state and CDobs is the signal at each data point in between N and D. Temperature scans were measured at (a) pH 8.0 and (b) at pH 5.5 and were fitted to a two-state unfolding model to obtain melting temperatures. Figure 5: Temperature-induced unfolding of NT E79QE119Q and NT E79QE84QE119Q . The CD signal was measured at 222 nm and converted to fraction folded according to the formula ([CD]obs–[CD]D)/([CD]N–[CD]D), where CD is the signal measured in mdegrees, CDD is the signal for the denatured state, CDN is the signal for the native state and CDobs is the signal at each data point in between N and D. Temperature scans were measured at ( a ) pH 8.0 and ( b ) at pH 5.5 and were fitted to a two-state unfolding model to obtain melting temperatures. Full size image Fluorescence cross-correlation spectroscopy (FCCS) We further investigated the monomer–dimer equilibrium of wt NT using FCCS. NT was labelled with either Atto488 or Cy5 fluorophores, attached through the addition of a cysteine residue at the N-terminus to allow site-specific maleimide coupling. The degree of labelling was determined with ESI-MS to be 70–80% for NT-Atto488 and 40–50% for NT-Cy5. Trp fluorescence showed identical dimerization behaviour for labelled proteins and unlabelled wt NT, with a 10-nm shift of the peak fluorescence intensity between pH 7 and 6 ( Supplementary Fig. 9 ). Measurement of the concentration of green–red dimers ‹ C GR › compared with the total concentration of green-labelled particles ‹ C G ›+‹ C GR › (see Methods) permitted the cross-correlated fraction to be plotted as a function of pH. FCCS analyses were performed on mixtures of NT-Atto488 and NT-Cy5 at 470 nM. Measurement of the cross-correlation from pH 7.3 to 5.2 revealed a p K a of dimerization at pH 6.1 and saturation, indicating a fully dimerized population, was reached below pH 5.5 ( Fig. 6 ). Upon measurement in the presence of 154 mM NaCl, the p K a of dimerization was not reached until around pH 5.5 and saturation was not established within the measured pH range ( Fig. 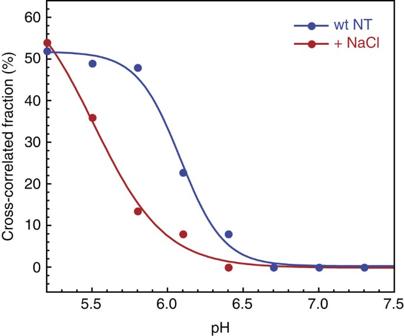6 ). Figure 6: The pKaof dimerization for wt NT measured with FCCS. Measured degree of dimer formation (cross-correlated fraction) versus pH, as determined by FCCS measurements. The relative degree of binding was determined from the measured concentration of green–red dimers (‹CGR› given by equation (13)) divided by the total concentration of green-labelled particles (‹CG›+‹CGR›, determined from equations (9–11)). In the dimerization process, also dimers will be formed, which consist of either two red-labelled or two green-labelled monomers. Moreover, since the fluorophore labelling efficiency is not 100% (70–80 and 40–50% for NT-atto488 and NT-Cy5, respectively) the FCCS measurements will not show complete dimerization. For wt NT in 20 mM HEPES/20 mM MES buffer (blue curve), the ratio ofreached a maximum plateau of about 50% for pH values below 5.5, which thus corresponds to full dimerization. For wt NT in the same buffer with 154 mM NaCl (red curve), the binding curve was shifted to lower pH, and a plateau/full dimerization could not be seen within the measured pH range. Calculating the dimerization byyields the same curves as shown in the figure but with different scaling of the amplitudes (data not shown). The solid line represents the equation from fitting the data to a two-state binding model and the results are representative of two experiments. Figure 6: The p K a of dimerization for wt NT measured with FCCS. Measured degree of dimer formation (cross-correlated fraction) versus pH, as determined by FCCS measurements. The relative degree of binding was determined from the measured concentration of green–red dimers (‹ C GR › given by equation (13)) divided by the total concentration of green-labelled particles (‹ C G ›+‹ C GR ›, determined from equations (9–11)). In the dimerization process, also dimers will be formed, which consist of either two red-labelled or two green-labelled monomers. Moreover, since the fluorophore labelling efficiency is not 100% (70–80 and 40–50% for NT-atto488 and NT-Cy5, respectively) the FCCS measurements will not show complete dimerization. For wt NT in 20 mM HEPES/20 mM MES buffer (blue curve), the ratio of reached a maximum plateau of about 50% for pH values below 5.5, which thus corresponds to full dimerization. For wt NT in the same buffer with 154 mM NaCl (red curve), the binding curve was shifted to lower pH, and a plateau/full dimerization could not be seen within the measured pH range. Calculating the dimerization by yields the same curves as shown in the figure but with different scaling of the amplitudes (data not shown). The solid line represents the equation from fitting the data to a two-state binding model and the results are representative of two experiments. Full size image The molecular mechanism now proposed involves a three-step process in which NT monomers first associate ( Fig. 7a,b ), and then form weakly associated dimers ( Fig. 7b,c ) that upon further lowering of the pH form stable dimers ( Fig. 7c,d ). We found evidence that during NT monomer to dimer conversion, multiple residues contribute to the proton uptake ( Fig. 7 ). A triple mutant NT E79QE84QE119Q mimics the behaviour of wt NT at low pH by forming a constitutive dimer over the whole pH range 5.0–7.5, as measured by Trp fluorescence spectroscopy ( Fig. 2a ), ESI-MS ( Supplementary Fig. 6 ) and HDX ( Supplementary Fig. 7 ). Furthermore, both at pH 5.5 and pH 7–8, the mutant shows similar thermal stability ( Fig. 5 ) and HSQC NMR spectrum ( Fig. 3 ) to the wt dimer at pH 5.5. Together, our data strongly support that E79, E84 and E119 are the titratable residues responsible for pH-dependent dimerization of NT. Contrastingly, removal of the charged side chains of D40, K65 and R60 stabilizes the monomer conformation, meaning that these residues remain charged and contribute to the stability of the dimer by intersubunit salt-bridge formation. In addition, they play a role in the electrostatic interactions leading to association of monomers ( Fig. 7a,b ), which result in the elevated pKa values for E79, E84 and E119 that enable protonation-induced dimerization and stabilization ( Fig. 7b–d ). E84 seems to have a dual role in monomer to dimer conversion. The single mutant NT E84Q promotes the monomer slightly ( Fig. 2a ), this is pronounced in the presence of salt ( Supplementary Fig. 5a ). Addition of the E84Q mutation to the NT E79QE119Q mutant, however, results in promotion of the dimer, giving a constitutive dimer that is similar to wt NT at pH 5.5. It appears that E84 (in its charged state) takes part in intersubunit charge interactions with R60/K65, together with the main determinant D40, thereby promoting association of monomers ( Fig. 7a,b ). This is supported by a significantly lower p K a of dimerization for the double mutant NT D40NE84Q compared with the single mutant NT D40N ( Fig. 2a ). Since E79Q and E119Q, but not E84Q, stabilize the dimer when analysed with Trp fluorescence, we conclude that protonation of E79 and E119 at pH 6.5 is required for the conformational relocation of W10 and formation of a weakly associated dimer ( Fig. 7b,c ). In addition, urea-induced denaturation experiments show that, while NT E79QE119Q becomes more stable at low pH, NT E79QE84QE119Q has a similar stability over the whole pH range 7.5–5.0 ( Fig. 2d ). This strongly suggests that protonation of E84 is related to the stability of the dimer. Hence, subsequent protonation of E84 does not contribute to additional conformational changes of W10 but is required for fully stable dimers to form ( Fig. 7c,d ), possibly by allowing the formation of a D40-K65 salt bridge. The consistency between the total charge reduction for the triple mutant and the maximum proton uptake for wt NT, as calculated from stability data ( Fig. 2f ), provides further evidence that protonation of E84, E79 and E119 is required for the monomer to stable dimer transition. However, the D40N mutation also leads to a significant effect, with 2.2 fewer protons taken up compared with the uptake of wt NT. We suggest that this observation is not directly connected to prevention of protonation of D40, but rather that the D40N mutation leads to a loss of the intersubunit electrostatic interactions, whereby monomer subunits should have a lower capacity to associate and the proton difference may then rather reflect reduced ability of E79 and E119 to protonate. A molecular dynamics simulation confirms that the p K a values of E79 and E119 are shifted to higher values in the dimer but not in the monomer [20] . Considering the close proximity of D40 and E84 in the dimer, the single mutation D40N may also result in a reduced ability for E84 to protonate due to a mutation-induced shift in p K a . This illuminates the need for simultaneous mutation of residues that may titrate in the same pH interval. E79, E84 and E119 are well conserved, E79 and E84 can be replaced by Asp and E119 can be replaced by a basic residue in some tubiliform spidroins. Moreover, D40, alongside with G110 is one of two strictly conserved residues [23] , [24] . This suggests that the charge network studied herein is representative for most NTs. The mutation D40N results in an inability to form dimers in the presence of NaCl at a pH as low as 5–5.5 ( Supplementary Fig. 5a ). This indicates that D40 may be conserved at least in part due to dimerization being essential for NT function. Intriguingly, the greatest proton difference is not reflected by monomer–dimer p K a but rather occurs for both wt NT and the mutants at around pH 5.7 ( Fig. 2e,f ). Furthermore, the transition point from urea stability data is at pH 5.6 for wt NT ( Fig. 2c ); this is one pH unit lower than the p K a of dimerization measured with Trp fluorescence. There seems to be an uncoupling between the conformational relocation of Trp10 and the formation of a fully stable dimer. In addition, FCCS analysis revealed a p K a of dimerization at pH 6.1 ( Fig. 6 ) with a fully dimerized population observed between pH 5.0 and 5.5, which coincides with the highest stability measured by urea denaturation. FCCS measures the correlated motion of fluorescent NT subunits—that is, the degree of binding, independently of conformational stages—and thus the p K a of dimerization measured by FCCS is expected to reflect the complete dimerization process. The divergence between stability data and Trp fluorescence data with an expected average measured by FCCS demonstrates that NT dimerization includes two distinct stages regulated by sequential protonation. We therefore suggest a novel dimerization mechanism that involves an intermediate stage of weakly associated dimers mediated by protonation of E79 and E119 ( Fig. 7c ), which become fully stabilized upon protonation of E84 at an even lower pH ( Fig. 7d ). Considering the spinning process in the duct of the spider silk gland, this mechanism appears biologically coherent. Since spider silk can be produced at a very high speed, the spidroins, including the NT domain, need to diffuse and associate at extremely high rates and/or pre-alignment of spidroins circumvent this requirement. From kinetic analysis of single NT mutants, it was recently suggested that NT dimerization between pH 7 and pH 6 indeed occurs by an unusually high association rate, which was suggested to facilitate fibre formation at a high reeling speed [21] . Our observations indicate that NT dimerization is a process that occurs over a much wider pH range, and the measured association rates may reflect only a part of this process. We propose that spiders have developed a mechanism by which NT monomers (i) associate by electrostatic interactions and (ii) at around pH 6.5 pre-align by forming weakly associated dimers, which still permit structural rearrangements of the spidroins and thereby safeguard against precocious assembly. Close to the exit point, the pH drops to 5.5 or below whereby (iii) NT forms stable dimers, interconnecting the spidroins, which allows the pulling forces in the fibre to be propagated via the protein chains, thereby facilitating the structural conversion of the repetitive parts. The already aligned, weakly associated dimers enable stable NT dimers to form very rapidly, since the process at this stage is independent of subunit association rate. Further studies are warranted to determine kinetic parameters for all steps underlying sequential NT dimerization. Site-directed mutagenesis of NT mutants The previously described vector pT7HisTrxHisNT [25] , containing the wt NT sequence, was subjected to point mutagenesis using the QuickChange site-directed mutagenesis kit (Agilent Technologies, Santa Clara, CA, USA) according to the manufacturer’s recommendations. Double and triple mutants were produced by consecutive point mutagenesis. After sequence verification, plasmids were digested with restriction enzymes EcoRI and HindIII to isolate DNA fragments containing only the mutated NT sequences. The fragments were purified on a 1 % agarose gel and ligated into pT7HisTrxHisNT, previously digested with the same enzymes to remove wt NT. The ligation mixtures were heat-shock-transformed into chemically competent Escherichia coli Nova Blue cells followed by plasmid preparation and sequence verification. Protein expression and purification The plasmids were heat-shock-transformed into chemically competent E. coli BL21 (DE3) cells before expression. For each variant, cells were inoculated to 10 ml Luria-Bertani medium with 70 mg l −1 kanamycin and grown overnight at 37 °C and 180 r.p.m. The overnight culture was used for a 1/100 inoculation of 500-ml Luria-Bertani medium with kanamycin. After growth at 37 °C to OD 600 of ~1, isopropyl β-D-1-thiogalactopyranoside was added to a final concentration of 0.5 mM followed by incubation at 30 °C for 4 h. The cells were harvested by centrifugation, resuspended in loading buffer (20 mM Tris-HCl, pH 8) and stored at −20 °C before purification. Lysis was performed on ice for 1 h in the presence of lysozyme and DNAse I, followed by centrifugation at 27,000 × g , 4 °C for 1 h. The cleared lysate was loaded to an IMAC column, previously packed with Ni-Sepharose and equilibrated with loading buffer. Bound protein was washed and eluted with loading buffer supplemented with 10 mM imidazole and 300 mM imidazole, respectively. Digestion with thrombin was performed during overnight dialysis in 5-l loading buffer, using a Spectra/Por dialysis membrane with a 6- to 8-kDa molecular weight cutoff. In order to remove the His-Trx-His tag, the sample was loaded to a Ni-Sepharose column as described, and unbound target protein was collected. The purity of the protein was determined by SDS–polyacrylamide gel electrophoresis using a 15% acrylamide gel stained with Coomassie Brilliant Blue. Tryptophan fluorescence measurements Fluorescence emission spectra were measured on a spectrofluorometer (Tecan Safire 2) using Costar black polystyrene assay plates with 96 flat bottom wells. The proteins were diluted to a concentration of 5 μM in 20 mM HEPES/20 mM MES adjusted to pH 5.6–7.4 in steps of 0.2 pH units. For experiments involving salt, the buffers were supplemented with NaCl, NaNO 3 or KCl at 154 mM or Na 2 SO 4 at 103 mM. The samples were excited at 280 nm using a 5-nm bandwidth, and emission spectra were recorded in 1 nm steps between 300 and 400 nm using a 10-nm bandwidth. The data were expressed as the ratio between the fluorescence at 339 and 351 nm as a function of pH and when possible fitted to a two-state binding model. Urea denaturation Urea-induced denaturation was performed by diluting the protein to 5 μM in 20 mM HEPES/20 mM MES with 0–7 M urea in 0.5 M steps. Trp fluorescence measurements were taken as described, at constant pH values ranging from 5.0 to 7.5 with 0.5 unit steps. For each measured pH, the fluorescence ratio was plotted against the urea concentration and fitted to a two-state unfolding model in order to determine the transition point. Calculation of proton uptake from urea denaturation data Wt NT and many of the mutants are dimeric in the lower end of this pH range and monomeric at the higher end. For the monomeric protein, unfolding can be analysed according to the model D↔N, where D is the denatured state and N is the native state. Using the standard assumption that the log of the equilibrium constant (log K D−N , where K D−N =[N]/[D]) is linearly proportional to the urea concentration [den] with a proportionality constant m D−N , we can analyse the data using the following equation [26] : where F is the measured signal, α N and α D are the signals of the native and denatured states in the absence of urea, β N and β D are the linear dependencies of these signals on [urea], and [den] 50% is the concentration at which the protein is 50% denatured. For the dimer, we assume that unfolding occurs according to the model N 2 ↔2D, so that the folded dimer dissociates to unfolded monomer. Under such circumstances, the free energy of unfolding Δ G D−N is dependent on protein concentration and can be described as Δ G D−N = RT ln[ P ] o +Δ G D−N o , where [ P ] o is the total protein concentration at the monomer level and Δ G D−N o is the stability at a reference concentration [27] . In practice, because the population of dimer titrates over the pH range 7.5–5.0, leading to the co-existence of shifting populations of dimers with folded and unfolded monomers, we have analysed the data for each mutant at each pH value according to a simple two-state unfolding scheme to obtain the apparent free energy of unfolding: Values of m D−N are associated with greater errors than [den] 50% , giving rise to greater scatter in the values of Δ G D−N water at different pH values. Furthermore, they did not show any systematic trend with pH; therefore, for each mutant we have calculated an average value of m D−N ( Supplementary Table 2 ), which we have used in equation (4). The average m D−N value calculated for each mutant is the numerical average of the individual m D−N values obtained for each mutant from denaturation curves carried out at different pH values. In all cases, these average values are based on at least five different denaturation curves. The pH dependence of Δ G D−N water is very informative, since it provides information about the number of protons bound to the denatured and native states, respectively, according to the following equation [28] : where Q D and Q N are the number of protons bound to the denatured and native states, respectively. The factor 2.3 is the conversion factor (ln(10)) from natural to base 10 logarithm (2.3 RT =1.36 kcal mol −1 ). Data are best fitted to a fourth-order polynomial (where x=pH): stability Δ G D−N (pH)= m 0+ m 1* x + m 2* x 2 + m 3* x 3 + m 4* x 4 . The differential function for this is: ESI-MS and HDX-MS Mass spectrometric characterization of NT and NT mutants was performed as described previously [15] . Briefly, deuteration buffers were prepared by freeze-drying 200 μl of 20 mM phosphate buffer, pH 5.5 or 7.5, followed by reconstitution in 200 μl D 2 O. Purified NT was diluted from phosphate-buffered stock solutions in deuterated phosphate buffer, pH 7.5 or 5.5, to a final protein concentration of 30 μM and a Deuterium content of 90%. Exchange was quenched by the addition of trifluoroacetic acid (TFA) to a final concentration of 0.1% and immediate freezing in liquid nitrogen. Protein was digested online in a Porozyme pepsin cartridge (Applied Biosystems, Foster City, CA, USA), and peptic peptides were trapped and desalted in a Waters Symmetry C 18 trap column (Waters, Milford, MA, USA). Digestion and desalting were carried out in a single step for 10 min. Peptides were then eluted in a single step and delivered to the mass spectrometer via a TaperTip emitter (Proxeon, Odense, Denmark). For ESI-MS analysis of NT dimerization, NT and NT mutants were diluted in 20 mM ammonium acetate, pH 7.5 or 5.5, to a final concentration of 30 μM, and introduced into the mass spectrometer using borosilicate needles (Proxeon). Spectra were acquired in positive-ion mode with a Waters Ultima API mass spectrometer (Waters) equipped with a Z-spray source. The source temperature was 80 °C, the capillary voltage was 2.5 kV for HDX-MS and 1.7 for ESI-MS analysis. The mass spectrometer was operated in single-reflector mode to achieve a resolution of 10,000 (full-width at half-maximum). The mass scale was calibrated using [Glu1]fibrinopeptide B for HDX-MS and horse heart myoglobin for ESI-MS analysis. Spectra were analysed using the Waters MassLynx V4.1 software package (Waters). CD spectroscopy Experiments were performed on a 410-model CD spectrometer (Aviv biomedical Inc., Lakewood, NJ, USA) using 300-μl cuvettes with a 1-mm path length. For all measurements, the proteins were diluted to 10 μM in 5 mM phosphate buffer at pH 5.5 or pH 8.0. Spectra were recorded from 260 to 185 nm at 25 °C, after heating to 95 °C and again at 25 °C after the samples were allowed to cool down. Temperature scans were measured at a wavelength of 222 nm by recording 1 °C steps in the temperature interval 25–95 °C and data were fitted to a two-state unfolding model. [ 15 N, 1 H]-HSQC NMR measurements For each mutant, an overnight culture was used for a 1/100 inoculation to 500 ml minimal medium M9 containing 15 N-labelled ammonium chloride and 70 mg l −1 kanamycin. The cells were grown overnight at 22 °C to an OD 600 of 1.4. The proteins were expressed and purified as described above. HSQC NMR spectra were acquired at 25 °C on a Varian Unity Inova 600-MHz NMR spectrometer equipped with an HCN cold probe. First, an NMR sample of 15 N-labelled protein in 20 mM sodium acetate, 20 mM NaCl, pH 5.5 buffer was prepared and a 2D [ 15 N, 1 H]-HSQC NMR spectrum was recorded. Afterwards, the same sample was dialysed against 20 mM sodium phosphate, 300 mM NaCl, pH 7.2 buffer using an Amicon Ultra-15 centrifugal filter device with a 3-kDa-molecular weight cutoff, and a second [ 15 N, 1 H]-HSQC NMR spectrum was recorded. The spectra were processed and analysed using Bruker Topspin 3.1 software. Fluorescence cross-correlation spectroscopy (FCCS) Mutagenesis was performed to introduce a cysteine residue at the N-terminus of wt NT in the vector pT7HisTrxHisNT, using the QuickChange site-directed mutagenesis kit (Agilent Technologies) according to the manufacturer’s recommendations. After sequence verification, the plasmid was transformed into E. coli BL21 (DE3) cells. The protein was expressed and purified as described above; now using degassed buffers to avoid oxidation of cysteine residues during purification. Directly before labelling, a 1-mg ml −1 (70 μM) protein solution in phosphate-buffered saline, pH 7.2, was reduced with a 50-fold molar excess of Tris-(2-carboxyethyl)phosphine hydrochloride for 1 h at room temperature. The thiol-reactive fluorophores maleimide-Atto488 and maleimide-Cy5 were used to separately label NT with either of the two fluorophores. For each labelling reaction, 1-mg maleimide–fluorophore was diluted in dimethyl sulfoxide to 20 mM and added to the reduced protein solution to an ~15-fold molar excess of the fluorophore. The sample was incubated for 2 h at room temperature and 4 h at 4 °C followed by the addition of a 100-fold molar excess of β-mercaptoethanol to terminate the reaction. Unbound fluorophores were removed by extensive dialysis using a Spectra/Por dialysis membrane with a 6- to 8-kDa molecular weight cutoff. The buffer was exchanged from phosphate-buffered saline to 40 mM HEPES, pH 7.5, by a stepwise reduction of the NaCl concentration during several days. NT-Atto488 and NT-Cy5 were stored separately at pH 7.3 to prevent binding. Before FCCS measurements, proteins labelled with different fluorophores were mixed and incubated for 30 min, followed by dilution in 20 mM HEPES/20 mM MES buffer, or the same buffer with 154 mM NaCl, at pH 5.2–7.3 with 0.3 unit steps. A home-built confocal setup comprising an Olympys IX-70 microscope body, an Ar-ion laser (Carl Zeiss, Jena, Germany, rebuilt by LASOS Laser-Fertigung GmbH, Jena, Germany) operated at 488 nm with excitation filter Z488/ × 10 (Chroma Technology Corp.) and a 594-nm He-Ne laser (Laser 2,000 GmbH), was used for the measurements. After reflection from a dichroic beam splitter Z488/594 (Chroma Technology Corp.), the laser beams were focused into the sample by an Olympus × 60, NA 1.2, UPlanApo objective. Fluorescence was collected by the same objective, separated from the excitation light and subsequently split into two wavelength ranges by a dichroic mirror, centred at 620 nm (620DCXR, Rockingham, VT, USA). Each of the spectrally separated emission light beams were imaged by a 150-mm achromatic lens onto a pinhole of 50 μm in diameter. Then, after re-collimation, each beam was focused into two avalanche photodiodes (SPCM-AQR-14, Perkin-Elmer Optoelectronics) in a beam-splitting arrangement. Two detectors were used in order to eliminate all influences of the inherent noise, detector’s ‘dead time’ and after pulsing effects. Rayleigh and Raman-scattered excitation light was suppressed by two band-pass filters, HQ532/70M and 690DF40 (Chroma Technology Corp. and Omega Optical Inc., Brattleboro, VT, USA, respectively), that were inserted in front of each detector. The signal from the photodiodes was analysed by an ALV-5000/E correlator (ALV-GmbH, Langen, Germany), with an ALV-5000/FAST Tau Extension board giving 12.5-ns lag time resolution when cross-correlating between channels. A detailed sketch of the setup has been previously described [29] . In FCS and FCCS, fluctuations in the detected fluorescence intensity F ( t ), generated by molecular diffusions through a focused laser beam (confocal detection volume) are analysed by: Here ‹ F i ( t )› and ‹ F j ( t )› are the time-averaged fluorescence signals of the fluorescence species i and j , and δF denotes their fluctuations around the mean at the times t and ( t + τ ). With i = j , equation (7) results in a single colour autocorrelation function: Here ‹ C › is the concentration of fluorescent molecules, Diff (τ)=(1+( ) −1 (1+( r 0 / z 0 ) 2 τ/τ D ) −1/2 denotes the temporal decay function of each diffusing species, τ D is the diffusion time through the detection volume, r 0 and z 0 are the structural parameters determined by the experimental geometry of the confocal detection volume V eff . With i ≠ j , equation (7) results in a two-colour cross-correlation function where [30] , [31] : Here indices G, R and GR correspond to green-only, red-only and green–red-labelled species, respectively. The number of double-labelled species can be determined by analysing both the cross and the autocorrelation functions recorded in the same experiment. The denominator of equation (11) can be expressed by the single colour autocorrelation amplitudes G GG (0) and G RR (0): Thus, the concentration of double-labelled species can be written as: In the calculation of <C GR > , cross-talk and a slight inevitable miss-match of the detection volumes of the red and green fluorescence signals were corrected for, as previously described [31] . NMR structure determination of wt NT at pH 5.5 A uniformly 13 C, 15 N-labelled sample of wt E. australis MaSp1 NT was prepared as previously described [16] . NMR experiments were performed at 298 K on a 600‐MHz Varian Unity Inova spectrometer equipped with an HCN triple‐resonance pulsed‐field‐gradient cold probe. The NMR sample of wt NT contained 1.5 mM protein, 20 mM sodium acetate (pH 5.5), 20 mM NaCl, 5% (v/v) D 2 O and 0.03% (w/v) NaN 3 . The following 2D and 3D spectra were recorded, with the number of complex points and mixing times as given in parenthesis: [ 15 N- 1 H]-HSQC (1,024 × 256), HNCA (1,024 × 32 × 64), 15 N-resolved NOESY-HSQC (1,024 × 38 × 150, 60 ms), 13 C(aliphatic)-resolved NOESY-HSQC (768 × 52 × 150, 60 ms) and 13 C(aromatic)-resolved NOESY-HSQC (1,024 × 48 × 128, 60 ms). All spectra were processed with Bruker TopSpin 3.1 and analysed in CARA [32] . The assigned chemical shifts have been deposited in the BioMagResBank (accession code 18480). Backbone and side chain chemical shift assignment was performed starting from the assignments of the wt NT monomer at pH 7.2 (ref. 16 ) and most assignments were easily transferrable by interactive analysis of the spectra. Automated peak picking of the three NOESY spectra was performed using UNIO-ATNOS/CANDID 2.0.2 (refs 33 , 34 ). Distance restraints were obtained from these peak lists using the internal NOE calibration procedure of CYANA 2.1 (ref. 35 ). No explicit torsion-angle or hydrogen bond restraints were used in the input. Structure calculations were performed using CYANA 2.1 (ref. 35 ) and involved seven iterations of automated NOE assignment with the routine CANDID [34] followed by a simulated annealing procedure starting from 100 random conformers that were annealed in 10,000 steps using torsion-angle dynamics. Unambiguous distance restraints including intermolecular restraints were obtained in the last cycle of this automated procedure. Initially, a monomeric structure was calculated, which showed high resemblance to the crystal dimer subunit. Subsequent manual inspection of the NOESY spectra allowed the identification of 19 unambiguous unique intermolecular contacts ( Supplementary Fig. 2 ) that were used as distance constraints with an upper limit of 5 Å in the following structure calculations. We also checked that these contacts were not present in the NOESY spectra of wt NT monomer at pH 7.2. The validity of this approach is exemplified by the fact that these manually imposed contacts are only a fraction of all intermolecular contacts established during automated NOE assignment and structure calculation. Although a calculation starting from random conformers converged to a dimer structure that was very similar to the crystal dimer, for the final structure calculation we additionally used the crystal structure as a model during the first cycle of the calculation to ensure better structural convergence. The 20 conformers ( Supplementary Fig. 10 ) with the lowest residual restraint violations were energy-minimized in a water shell using the program CNS 1.2 (refs 36 , 37 ) and their coordinates were deposited in the PDB (accession code 2LTH). Structure quality and goodness-of-fit to the NMR data were evaluated using RPF scores [22] . Supplementary Table 1 shows an overview of the restraints used and structural statistics. Ramachandran statistics: 92.0% most favoured, 7.4% additionally allowed, 0.5% generously allowed and 0.1% disallowed regions. How to cite this article: Kronqvist, N. et al . Sequential pH-driven dimerization and stabilization of the N-terminal domain enables rapid spider silk formation. Nat. Commun. 5:3254 doi: 10.1038/ncomms4254 (2014).